Molecular basis of the alternative recruitment of GABAAversus glycine receptors through gephyrin γ-Aminobutyric acid type A and glycine receptors (GABA A Rs, GlyRs) are the major inhibitory neurotransmitter receptors and contribute to many synaptic functions, dysfunctions and human diseases. GABA A Rs are important drug targets regulated by direct interactions with the scaffolding protein gephyrin. Here we deduce the molecular basis of this interaction by chemical, biophysical and structural studies of the gephyrin–GABA A R α3 complex, revealing that the N-terminal region of the α3 peptide occupies the same binding site as the GlyR β subunit, whereas the C-terminal moiety, which is conserved among all synaptic GABA A R α subunits, engages in unique interactions. Thermodynamic dissections of the gephyrin–receptor interactions identify two residues as primary determinants for gephyrin’s subunit preference. This first structural evidence for the gephyrin-mediated synaptic accumulation of GABA A Rs offers a framework for future investigations into the regulation of inhibitory synaptic strength and for the development of mechanistically and therapeutically relevant compounds targeting the gephyrin–GABA A R interaction. γ-Aminobutyric acid type A receptors (GABA A Rs) are ligand-gated ion channels, which mediate the majority of fast inhibitory synaptic transmission in the mammalian central nervous system. Deficits in GABA A R-mediated neurotransmission have been implicated in a wide spectrum of disorders of the central nervous system, such as epilepsy, anxiety, mood disorders and neuro-developmental impairments including autism, fragile X syndrome and schizophrenia [1] . Accordingly, GABA A Rs are important, validated drug targets and compounds targeting GABA A Rs have been extensively explored and successfully used clinically as sedatives, anxiolytics and anticonvulsive drugs, narcotics and anaesthetics, anti-spasmodics, anti-epileptics, hypnotic and analgesic drugs. GABA A Rs are pentameric hetero-oligomers assembled from seven different subunit classes with the most common receptor combination being two α, two β and a single γ subunit [2] . The majority of synaptic GABA A R subtypes are localized and accumulated by the scaffolding protein gephyrin. Gephyrin is a central player at inhibitory synapses and, besides the structural role as a receptor scaffold, gephyrin also acts as a platform for additional protein–protein interactions, bringing receptors, cytoskeletal elements and signalling proteins into close spatial proximity [3] , [4] , [5] . Therefore, insights into the molecular basis of GABA A R clustering at synaptic sites might allow the advance of new therapeutic principles in the treatment of GABA A R-related disorders. Gephyrin is composed of an N-terminal domain (GephG, residues 1–181) and a C-terminal domain (GephE, residues 318–736), which are connected by an unstructured linker (residues 182–317). Gephyrin was discovered [6] by co-purification with glycine receptors (GlyRs) and found to be responsible for anchoring and accumulating GlyRs at postsynaptic sites, which is accomplished by the simultaneous binding of gephyrin to the GlyR β subunit [7] , [8] , [9] , [10] and elements of the cytoskeleton [11] , [12] . A number of gene knockout studies have addressed the role of the gephyrin–GABA A R interaction in vivo . Gephyrin knock-out mice die within hours after birth [13] and analysis of these mice revealed a loss of GlyR clusters [13] and a subset of GABA A R clusters [14] . Similarly, gene knockouts of single GABA A R subunits, such as the γ2 and α3 subunit, not only interfere with GABA A R but also with gephyrin clustering [15] , [16] , [17] . An X-ray crystal structure of GephE in complex with a 49-residue peptide derived from the large cytoplasmic loop of the GlyR β subunit defined the gephyrin–GlyR interaction in atomic detail [10] . Recently, we demonstrated that the same region of gephyrin can act as a universal receptor-binding site [18] , which also mediates the interactions with the GABA A R α1, α2 and α3 subunits [19] , [20] , [21] , and that this interaction is modulated by the oligomeric state of gephyrin together with the number of receptor-binding subunits [22] , possibly explaining the extremely slow exchange rates of GlyRs at synaptic sites [23] . Recent studies have highlighted the critical role of the GABA A R α subunits in gephyrin-mediated synaptic versus extrasynaptic targeting of GABA A Rs, which has been verified in cell-based, electrophysiological [24] and immunohistochemical experiments [14] , [19] , [20] , [21] . Despite its fundamental function in synaptic receptor localization ( Fig. 1 ), receptor diffusion dynamics [20] and synaptic plasticity [25] , the gephyrin–GABA A R interaction has not yet been elucidated on the molecular level. In this study, we describe the crystal structure of a gephyrin–GABA A R complex and identify key residues in gephyrin and the GABA A Rs that drive the gephyrin-mediated recruitment of GABA A Rs to postsynaptic sites. This will allow for a rational approach to develop compounds that could perturb the gephyrin–GABA A R interaction, which will be of great mechanistic and pharmacological interest and could pave the way for new approaches in targeting GABA A Rs in drug development. 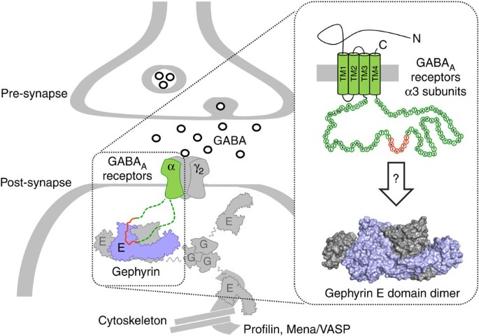Figure 1: Schematic view of a GABAergic synapse. Ionotropic γ-aminobutyric acid type A receptors (GABAARs) are pentameric membrane receptors that are clustered at synaptic sites by direct interactions with the anchoring protein gephyrin. Gephyrin is believed to form higher oligomers at synaptic sites by homotrimerization of its G domain and homodimerization of its E domain. Eleven residues, which are conserved among the synaptic GABAAR α subunits, directly engage with the E domain (PDB entry 4PD0) near the dimer interface (boxes). Gephyrin binding tethers the receptors to the cytoskeleton by direct interaction with profilin and Mena/VASP. Figure 1: Schematic view of a GABAergic synapse. Ionotropic γ-aminobutyric acid type A receptors (GABA A Rs) are pentameric membrane receptors that are clustered at synaptic sites by direct interactions with the anchoring protein gephyrin. Gephyrin is believed to form higher oligomers at synaptic sites by homotrimerization of its G domain and homodimerization of its E domain. Eleven residues, which are conserved among the synaptic GABA A R α subunits, directly engage with the E domain (PDB entry 4PD0) near the dimer interface (boxes). Gephyrin binding tethers the receptors to the cytoskeleton by direct interaction with profilin and Mena/VASP. Full size image Identification of GABA A R α3-derived minimal peptides Previous attempts to structurally characterize the interactions between GephE and the full-length intracellular loops of the GABA A R α1, α2 and α3 subunit were hampered by the low affinities and low solubility of the isolated loop regions. Accordingly, a primary challenge was to identify GABA A R-derived peptides appropriate for crystallization. The α3 subunit was selected as a template as it displays the highest in vitro gephyrin affinity of all GABA A R subunits with a K D of 5.3 μM for the full-length intracellular loop [18] , [20] , [21] , [26] . GABA A Rs containing α3 subunits co-localize with gephyrin in the cerebellar cortex [27] , thalamic reticular nucleus [17] and at perisomatic synapses in the globus pallidus [28] , and a knock-out of the α3 subunit results in disruption of postsynaptic gephyrin clusters [16] , [17] . In addition, structural insights into the gephyrin-α3 interaction would allow one to predict the interactions with the α1 and α2 subunits to gephyrin, as the binding motifs of these α subunits are conserved [18] . Based on the conserved N-terminal gephyrin-binding motif (FS/NIVG) in the GlyR β and GABA A R α3 subunits [18] , respectively, we synthesized a 20-residue GABA A R α3 fragment (referred to as α20, 367 TFNIVGTTYPINLAKDTEFS 386 ). However, the affinity of this 20-mer peptide was too low to be assessed by isothermal titration calorimetry (ITC) [18] . Hence, we first used peptide SPOT synthesis to perform a complete Ala-scan of the α20 peptide to characterize the molecular details of the GephE–GABA A R α3 interaction. For this assay, GephE was recombinantly expressed, purified and conjugated to horseradish peroxidase (HRP) to allow tracking of its peptide binding by chemiluminescence with high sensitivity. Fourteen different alanine mutants of the α20 peptide were immobilized in high density on a cellulose-based microarray (Celluspot, Intavis). After incubation with GephE-HRP, the chemiluminescence was quantified for each alanine mutant. We observed that Ala substitutions of residues 368–372 as well as 375 significantly impaired binding to GephE, whereas Ala substitutions of Thr373 and, in particular, Thr367 resulted in an increased binding affinity ( Fig. 2a ). 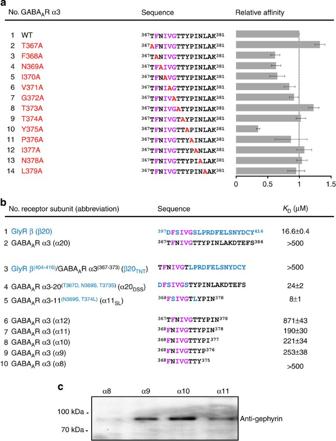Figure 2: Identification of short GABAAR-derived peptides as gephyrin-binding probes. (a) Peptide-array-based alanine-scan of the gephyrin core-binding site within the GABAAR α3 subunit. Residues shown in pink are conserved in the GABAAR α3 and GlyR β subunits. Gephyrin binding to peptides was detected by chemiluminescence of conjugated horseradish peroxidase. Shown are the relative averaged intensities of six peptide sets together with their standard deviations (error bars). Notably, T367A and T374A increase the gephyrin affinity, whereas an alanine exchange of residues 368–373 as well as residue 376 reduces gephyrin binding. (b) ITC analysis of gephyrin binding to GABAAR α3 and GlyR β/GABAAR α3 chimeric peptides. Peptide sequences and respective GephE affinities are shown. Peptides containing the seven N-terminal residues of the GlyR β peptide display a potentiated gephyrin affinity. N-terminal elongation reduces the affinity, whereas C-terminal elongation has an affinity-enhancing effect. (c) Short GABAAR-derived peptides were sufficient to retain native gephyrin. Pull-down of native gephyrin from whole mouse brain lysate using immobilized short GABAAR-derived peptides. Immunedetection of gephyrin reveals that peptides with a length of 9–11 residues (α9-α11) were sufficient for gephyrin binding, whereas an octamer (α8) did not display binding. The complete blot is shown inSupplementary Fig. 1. Figure 2: Identification of short GABA A R-derived peptides as gephyrin-binding probes. ( a ) Peptide-array-based alanine-scan of the gephyrin core-binding site within the GABA A R α3 subunit. Residues shown in pink are conserved in the GABA A R α3 and GlyR β subunits. Gephyrin binding to peptides was detected by chemiluminescence of conjugated horseradish peroxidase. Shown are the relative averaged intensities of six peptide sets together with their standard deviations (error bars). Notably, T367A and T374A increase the gephyrin affinity, whereas an alanine exchange of residues 368–373 as well as residue 376 reduces gephyrin binding. ( b ) ITC analysis of gephyrin binding to GABA A R α3 and GlyR β/GABA A R α3 chimeric peptides. Peptide sequences and respective GephE affinities are shown. Peptides containing the seven N-terminal residues of the GlyR β peptide display a potentiated gephyrin affinity. N-terminal elongation reduces the affinity, whereas C-terminal elongation has an affinity-enhancing effect. ( c ) Short GABA A R-derived peptides were sufficient to retain native gephyrin. Pull-down of native gephyrin from whole mouse brain lysate using immobilized short GABA A R-derived peptides. Immunedetection of gephyrin reveals that peptides with a length of 9–11 residues (α9-α11) were sufficient for gephyrin binding, whereas an octamer (α8) did not display binding. The complete blot is shown in Supplementary Fig. 1 . Full size image In an attempt to increase the affinity of the GABA A R-derived binding peptide and to map differences in the way GABA A R and GlyR interact with gephyrin, we designed and prepared GABA A R α3/GlyR β chimeric peptides and quantified their binding affinity by ITC ( Fig. 2b ). We found that the affinity of the α20 peptide could be increased by substituting seven N-terminal residues with those derived from the GlyR β subunit ( Fig. 2b , sequences no. 4 and 5), whereas substitution with 13 C-terminal residues from GlyR β did not lead to detectable changes in affinity ( Fig. 2b , sequence no. 3). Based on the Ala-scan and chimeric peptides, we then synthesized optimized variants of GABA A R α3-derived peptides corresponding to the N-terminal region of the GlyR β gephyrin-binding site lacking the N-terminal Thr367 ( Fig. 2b , sequences no. 5–10). Strikingly, three GABA A R α3 subunit peptide fragments varying in length from 9 to 11 residues (referred to as α9–11) displayed a micromolar affinity to GephE in ITC experiments ( Fig. 2b , sequences no. 7–9). This correlates with the Ala-scan showing that the Thr367Ala mutation increased affinity to GephE ( Fig. 2b ), and this possibly explains why gephyrin binding of longer GABA A R-derived synthetic peptides could not be quantified by ITC earlier [18] . Thus, we identified short and soluble GABA A R α3-derived peptides, α9–11, exhibiting micromolar affinity to GephE, which was essential for our overall aim of delineating the gephyrin–GABA A R interaction. Short GABA A R α3-derived peptides bind native gephyrin Phosphorylation [29] , [30] , [31] , [32] , palmitoylation [33] , [34] and acetylation [35] , [36] of gephyrin have been reported and these post-translational modifications have been shown to affect the structure, trafficking, half-life and importantly the ability of gephyrin to interact with partner proteins. To test whether the identified short GABA A R-derived peptide fragments α9–11 also mediate binding to native full-length gephyrin comprising post-translational modifications, the peptides were covalently immobilized on iodoacetyl-activated beads and subsequently incubated with mouse brain lysates. In accordance with the recombinant GephE-based ITC results, α9–11 peptides, but not α8, could retain wild-type gephyrin on the beads, which was verified using the phosphospecific antibody mab7a [37] ( Fig. 2c and Supplementary Fig. 1 ). Thus, the identified peptides not only bind to GephE in vitro , but also to full-length wild-type gephyrin from adult mouse brain. Crystal structures of GephE in complex with GABA A R α3 fragments Co-crystallization trials with GephE in combination with either the medium-affinity α11 WT peptide (FNIVGTTYPIN) or the high-affinity α11 SL peptide (FNIVGSLYPIN) yielded four co-crystal structures belonging to two crystal forms ( Table 1 ): (i) hexagonal crystals (space group P6 1 ), which were previously described for the GephE-GlyR complex [38] , diffracting to resolutions of 3.6 and 4.1 Å ( Supplementary Fig. 2 and Table 1 ). (ii) Orthorhombic crystals (space group P2 1 2 1 2) diffracting to 2.7 Å resolution ( Figs 3 and 4 , Supplementary Fig. 3 and Table 1 ), which were related to GephE-GlyR and apo-GephE structures [10] , [22] . The α11 WT and α11 SL peptides were clearly defined in the electron density maps ( Fig. 3c and Supplementary Figs 4 and 5 ) in both crystal forms, allowing us to model either all or the first nine residues of the 11-mer GABA A R peptide fragment ( Figs 3 and 4 and Supplementary Fig. 2 ). Table 1 Data collection and structure refinement. 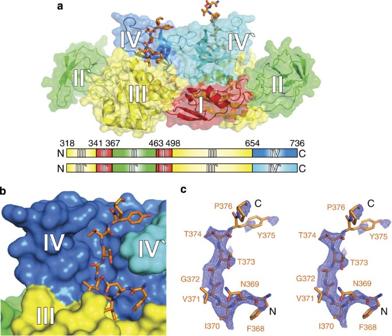Figure 3: X-ray crystal structure of GephE in complex with the GABAAR α3 peptide fragment. (a)Cartoon representation of GephE in complex with the GABAAR α3-derived peptide α11WT(PDB-ID: 4TK1) colour-coded according to its subdomain architecture as indicated (scheme at the bottom). The residues of α11WTresolved in the structure (368FNIVGTTYP376) are shown as a stick model in orange. (b) Close-up view into the binding pocket. Surface representation of the GephE-binding pocket coloured according toa. The GABAAR peptide is tightly packed into the cleft formed by subdomains III and IV from one monomer, as well as subdomain IV′ from the other monomer. (c)Fo−Fcomit electron density map of the GABAAR α3 peptide (stereo representation) contoured at an rms deviation of 2.5 in blue with the modelled peptide in stick representation. Full size table Figure 3: X-ray crystal structure of GephE in complex with the GABA A R α3 peptide fragment. (a) Cartoon representation of GephE in complex with the GABA A R α3-derived peptide α11 WT (PDB-ID: 4TK1) colour-coded according to its subdomain architecture as indicated (scheme at the bottom). The residues of α11 WT resolved in the structure ( 368 FNIVGTTYP 376 ) are shown as a stick model in orange. ( b ) Close-up view into the binding pocket. Surface representation of the GephE-binding pocket coloured according to a . The GABA A R peptide is tightly packed into the cleft formed by subdomains III and IV from one monomer, as well as subdomain IV′ from the other monomer. ( c ) F o − F c omit electron density map of the GABA A R α3 peptide (stereo representation) contoured at an rms deviation of 2.5 in blue with the modelled peptide in stick representation. 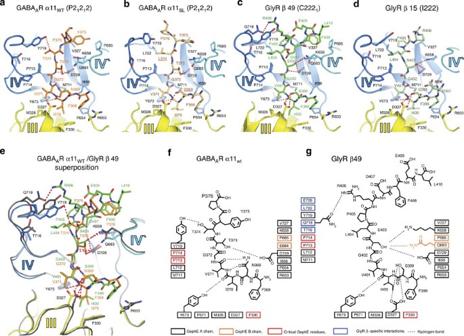Figure 4: Molecular details of subunit-specific gephyrin interactions. Close up view of the interactions between GephE with (a) GABAAR α3 wild-type-derived peptide (PDB-ID 4TK1), (b) α11SLpeptide (PDB-ID 4TK3) and (c,d) GlyR β-derived peptides (PDB-ID 2FTS10and 4PD1 (ref.22)) as well as (e) a superposition and (f,g) schematic 2D representations of the GlyR β wild-type and GABAAR α3 wild-type interactions. Ina–d, residues mediating the interactions are highlighted in stick representation and are numbered (coloured for the peptides, black for GephE). GephE residues located in subdomain III are coloured in yellow, residues from subdomain IV in marine blue and GephE residues derived from the other subdomain IV′ in cyan. Hydrogen bonds are shown as dotted red lines. Note that the N-terminal-binding motifs engage in conserved interactions, whereas the C-terminal halves interact differentially with GephE. Full size image Figure 4: Molecular details of subunit-specific gephyrin interactions. Close up view of the interactions between GephE with ( a ) GABA A R α3 wild-type-derived peptide (PDB-ID 4TK1), ( b ) α11 SL peptide (PDB-ID 4TK3) and ( c , d ) GlyR β-derived peptides (PDB-ID 2FTS [10] and 4PD1 (ref. 22 )) as well as ( e ) a superposition and ( f , g ) schematic 2D representations of the GlyR β wild-type and GABA A R α3 wild-type interactions. In a – d , residues mediating the interactions are highlighted in stick representation and are numbered (coloured for the peptides, black for GephE). GephE residues located in subdomain III are coloured in yellow, residues from subdomain IV in marine blue and GephE residues derived from the other subdomain IV′ in cyan. Hydrogen bonds are shown as dotted red lines. Note that the N-terminal-binding motifs engage in conserved interactions, whereas the C-terminal halves interact differentially with GephE. Full size image The GABA A R α3 and GlyR β-binding sites overlap significantly The crystal structures of GephE in complex with the GABA A R α3-derived peptide fragments revealed ( Fig. 3a ) that GephE is present as a homodimer with each subunit consisting of four subdomains as described previously [10] , [22] , [38] . The GephE dimer is in complex with two symmetrically arranged receptor fragments ( Fig. 3a ), where subdomains III and IV of one GephE monomer as well as subdomain IV of a second monomer (IV′) together from a common receptor-binding site ( Figs 3 and 4 ) for peptides derived from either the GABA A R α3 or the GlyR β subunit [10] , [22] , [38] . The interactions of the peptides derived from either receptor with subdomain III are nearly identical, whereas the interactions with subdomain IV and IV′ are receptor specific ( Fig. 4 and Supplementary Fig. 2 ). GABA A R α3 and GlyR β also engage in receptor-specific interactions A direct comparison of the two GephE-α11 WT structures with the two GephE-α11 SL structures ( Fig. 4a,b and Supplementary Fig. 2a,b ) as well as the corresponding GlyR β structures ( Fig. 4c,d ) [10] , [22] revealed distinct interactions with either receptor ( Fig. 4e–g ). Based on the largely identical N-terminal interactions for α11 WT - and GlyR β-derived peptides, we defined the critical N-terminal aromatic residue, which is conserved in all gephyrin-binding receptor-derived peptides as position 1 (Phe368 in GABA A R α3, Phe398 in GlyR β) and based on previous mutational studies [18] this residue corresponds to Tyr340 in GABA A R α1 and Tyr339 in GABA A R α2. The main chains of the conserved N-terminal residues (positions 1–7: GABA A R α3 368 FNIVGTT 374 , GlyR β 398 FSIVGSL 404 (refs 10 )) adopted highly similar conformations ( Fig. 4e ), whereas their side chains formed subunit-specific interactions with gephyrin ( Fig. 4e ). The central four-stranded β-sheet of GephE subdomain IV and the first α-helix and several neighbouring residues of subdomain III engaged in identical interactions with the peptides from either the GABA A R α3 or GlyR β subunits (positions 1–5 corresponding to GABA A R 368 FNIVG 372 and GlyR 398 FSIVG 402 ), with the exception of position 2 (Asn369 in GABA A R, Ser399 in GlyR). Notably, the hydrogen-bonded interactions of GABA A R Asn369 with GephE Asp327 appeared to be less optimal when compared with the corresponding hydrogen bonds of Ser399 in GlyR β, thereby contributing to the lower affinity of the GABA A R. The subsequent residues of the GABA A R and GlyR loops (positions 6–7, GABA A R 373 TT 374 , GlyR 403 SL 404 ) interacted with gephyrin differently: GlyR β Ser403 forms additional hydrogen bonds compared with GABA A R Thr373 and, in addition, GABA A R Thr374 could not engage as efficiently with the large hydrophobic pocket formed by Thr716, Tyr719 and Leu722 of gephyrin compared with the corresponding Leu404 in the GlyR β subunit. The C-terminal residues (positions 8–11: GABA A R 375 YPIN 378 , GlyR 405 PRDFEL 410 ) differed substantially in both their side chain interactions and main chain conformations. Nonetheless, GABA A R α3 Tyr375 at position 8 mediates contacts to roughly the same hydrophobic interface on the second GephE monomer as GlyR β Phe408 at position 11. Remarkably, the elongated 49 residue GlyR β loop (β49) forms a short α-helical element, whereas the GABA A R-derived peptides displayed no secondary structure, and, as a result, the overall GephE–GlyR β-binding interface is significant larger (991 Å 2 ) than the corresponding GephE–GABA A R α3-binding interface (835 Å 2 ; Supplementary Tables 1 and 2 ). This may additionally contribute to the reduced affinity of GABA A R α3 to gephyrin compared with GlyR β. Thermodynamic dissection of the receptor specificity of gephyrin Based on the gephyrin-GABA A R α3 X-ray crystal structures, we designed and synthesized a range of point mutated GABA A R α3 peptide fragments and determined the thermodynamic basis of their gephyrin binding by ITC ( Fig. 5 ). Between the structurally resolved GABA A R ( 368 F N IVG TTYPIN 378 ) and GlyR ( 398 F S IVG SLPRDFEL 410 ) fragments, only the four underlined residues are conserved ( Fig. 5a ). Three of seven non-conserved residues are located at the C-terminal end (GABA A R 376 PIN 378 , GlyR 406 RDF 408 ), which is the region where the primary structural differences are found. Nonetheless, exchange of these residues between peptides derived from either GABA A R or GlyR did not alter the overall binding affinity significantly ( Fig. 5a ), thus indicating comparable binding contributions. Among the four remaining receptor subunit-specific residues, position 2 (GABA A R α3 Asn369, GlyR β Ser399) is located within the conserved N-terminal motif, which mediates the mutually exclusive receptor binding to gephyrin. ITC measurements verified the structural evidence ( Fig. 4a–d ); Ser399 could engage in more optimal hydrogen-bonding interactions with GephE compared with Asn369. The exchange of Ser399 with an Asn369 in GlyR resulted in an at least threefold reduced affinity (8.3±0.1 to 25.5 μM), vice versa, introduction of Ser for Asn369 in GABA A R increased the affinity at least sixfold (190±30 to 33±6 μM; Fig. 5a ). The three remaining subunit-specific residues were located near the centre of the receptor peptide fragments (positions 6–8, GABA A R 373 TTY 375 , GlyR 403 SLP 405 ). The ITC analysis revealed that both, the Ser403Thr and the Pro405Tyr exchange, enhanced the peptide fragment affinity (8.3±0.1 to 5.9±0.1 and 8.3±0.1 to 4.3±0.3 μM, respectively), and that this effect was based on additional hydrophobic interactions as reflected by the larger contribution of the entropy term to the overall affinity ( Fig. 5a ). Exchange of GlyR Leu404 with the corresponding GABA A R Thr reduced the GlyR affinity twofold (8.3±0.1 to 15.9±0.7 μM). In contrast, the corresponding exchange yielded a fivefold higher affinity (190±30 to 36±10 μM) for the GABA A R accompanied by a gain in entropy. This finding was in line with the additional hydrophobic interactions as indicated by the structural analysis ( Fig. 4a–d ). Remarkably, at position 8, the GlyR and the GABA A R subunit engaged in critical, yet different hydrophobic interactions, with either a Pro in case of the GlyR β subunit or a Tyr in the GABA A R α3 subunit. The critical nature of this ligand position was demonstrated by the corresponding Pro-to-Ala variant, which showed an at least sevenfold reduced affinity (8.3±0.1 to 62±24 μM; Fig. 5a ), in line with a loss of a large hydrophobic contact area as indicated by the crystal structure. Finally, a double mutation at positions 2 and 7 within both receptor peptide fragments reduced the GlyR fragment affinity 6-fold (8.3±0.1 to 47±19) and improved the GABA A R fragment affinity 25-fold (190±30 to 7.9±1.3 μM), yielding in the latter case an affinity identical to the GlyR fragment (8.3±0.1 μM; Supplementary Fig. 6 ). Thus, the ITC experiments provide a detailed picture of the thermodynamic basis of the subunit-specific gephyrin interactions. Together with the X-ray crystal structures, the thermodynamic data complete the picture of how GABA A Rs and GlyRs are recruited alternatively to postsynaptic sites by engaging with gephyrin as summarized in Fig. 5b . 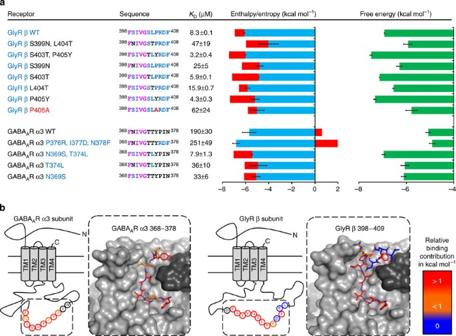Figure 5: Thermodynamic dissection of the subunit specificity of gephyrin. (a) Different contributions of the binding enthalpy and entropy to the overall free energy. Residues conserved among the GlyR β and GABAAR α3 subunits are shown in magenta, GlyR β residues in blue and GABAAR α3 residues in black. The GlyR β peptide displayed a 23-fold higher affinity than the corresponding GABAAR peptide. Subunit specific residues were exchanged between both receptor subunits. Note that the gephyrin affinity can be maximized by combining hydrophobic residues of GlyRs and GABAARs (GlyR S403T and GABAAR P405Y). Remarkably, full GlyR-like binding affinity can be reconstituted for the GABAAR fragment by only two mutations, N369S and T374L. Enthalpy, entropy and free energy bar graphs are averages (with their standard deviations indicated by the error bars) of at least three ITC measurements. (b) Differential binding of GABAARs and GlyRs to an overlapping gephyrin-binding site. Structures of the GlyR and GABAAR peptides in stick representation colour-coded according to the relative binding contribution (high (>1 kcal mol−1) in red, low (<1 kcal mol−1) in orange and none (~0 kcal mol−1) in blue) with the gephyrin surface shown in grey. The corresponding sequences of the full-length intracellular loops of GABAAR α3 and GlyR β are shown below using the same colour code. Note that different ligand residue positions mediate the critical gephyrin interactions. Figure 5: Thermodynamic dissection of the subunit specificity of gephyrin. ( a ) Different contributions of the binding enthalpy and entropy to the overall free energy. Residues conserved among the GlyR β and GABA A R α3 subunits are shown in magenta, GlyR β residues in blue and GABA A R α3 residues in black. The GlyR β peptide displayed a 23-fold higher affinity than the corresponding GABA A R peptide. Subunit specific residues were exchanged between both receptor subunits. Note that the gephyrin affinity can be maximized by combining hydrophobic residues of GlyRs and GABA A Rs (GlyR S403T and GABA A R P405Y). Remarkably, full GlyR-like binding affinity can be reconstituted for the GABA A R fragment by only two mutations, N369S and T374L. Enthalpy, entropy and free energy bar graphs are averages (with their standard deviations indicated by the error bars) of at least three ITC measurements. ( b ) Differential binding of GABA A Rs and GlyRs to an overlapping gephyrin-binding site. Structures of the GlyR and GABA A R peptides in stick representation colour-coded according to the relative binding contribution (high (>1 kcal mol −1 ) in red, low (<1 kcal mol −1 ) in orange and none (~0 kcal mol −1 ) in blue) with the gephyrin surface shown in grey. The corresponding sequences of the full-length intracellular loops of GABA A R α3 and GlyR β are shown below using the same colour code. Note that different ligand residue positions mediate the critical gephyrin interactions. Full size image Despite its fundamental importance for the function of the inhibitory synapse, the interactions with gephyrin that mediate the anchoring and accumulation of synaptic GABA A Rs were poorly understood. To address this, we designed GABA A R α3-derived gephyrin-binding peptides, which enabled the structural analysis of the gephyrin–GABA A R complex and revealed how GABA A Rs containing the α3 subunit are clustered at synaptic sites. Despite their binding to an overlapping site in the gephyrin protein compared with GlyRs, GABA A Rs engage in subunit-specific interactions allowing for an alternative recruitment of inhibitory receptors by gephyrin. In addition, our study identifies two residues (GlyR β Ser399 and Leu404 vs. GABA A R α3 Asn369 and Thr374) as major determinants for gephyrin’s distinct preference for the GlyR β subunit over the GABA A R α3 subunit. Thus, we have provided the structural basis for the mutually exclusive binding of GABA A R and GlyR to the scaffold protein gephyrin [18] . Here we present the structural and thermodynamic analysis of gephyrin binding to short peptides, either native to the GABA A R α3 subunit or rationally designed. Notably, the full-length intracellular loop of GABA A R α3 displays an enhanced affinity ( K D =5.3 μM) [18] , [21] compared with the truncated α11 WT variant ( K D =190 μM) analysed here. The 11mer mediates ~70% of the free energy and ~86% of the enthalpy compared with the GABA A R α3 full-length intracellular loop [21] when interacting with gephyrin. Although the molecular basis of the enhanced binding cannot be fully explained, the beneficial entropic contribution of the full-length fragment suggests that secondary and/or tertiary structure effects in the full-length intracellular loop present the core-binding site in a more favourable orientation and are thus responsible for its stronger binding. Furthermore, the α11 WT peptide ( 368 FNIVGTTYPIN 378 ) occupies an overlapping binding site ( Fig. 4e ) compared with the GlyR fragment resolved earlier ( 398 FSIVGSLPRDFELS 411 ), which, in turn, could be used to completely block gephyrin binding of GABA A R-derived full-length intracellular loops [18] . In addition, single point-mutations within the core region of the α3-derived peptide ( 368 FNIVGTTY 375 ) were shown [18] to completely abolish gephyrin binding of the full-length loop and, vice versa, loops missing the core motif were demonstrated to completely lose their ability to mediate receptor clustering in neurons or to mediate binding in yeast two-hybrid experiments [21] . Taken together, it can be concluded that the remainder of the intracellular loop exerts a critical enhancing effect, but does not provide a second independent binding site that would be sufficient for binding in primary hippocampal neurons, yeast two-hybrid, ITC or pull-down assays. A direct comparison of the gephyrin affinity to the core-binding sites of GlyR and GABA A R confirmed an approximately 25-fold preference of gephyrin for GlyRs containing the β subunit over GABA A Rs containing the α3 subunit. The structural and thermodynamic mutational analysis revealed that Ser399 of the GlyR binds more effectively than the corresponding Asn369 in the GABA A R α3 subunit, whereas Leu404 of the GlyR creates a larger hydrophobic binding interface than the corresponding GABA A R α3 residue Thr374 ( Fig. 4 and Supplementary Fig. 6 ). Together, the slight differences in the side chain interactions synergistically result in the distinct subunit preference of gephyrin for GlyRs over α3-containing GABA A Rs. Gephyrin mediates GABA A R α3 and GlyR β binding via a large groove formed by subdomains III and IV ( Fig. 3b ) within GephE. The N-terminal part of the receptor core-binding sites relies on highly conserved receptor interactions and involves hydrophobic contacts between Phe330 of gephyrin and the respective aromatic residues in the receptors, but also critical hydrogen bonds mediated by Tyr673 and Asp327 of gephyrin. We observed that the seven N-terminal residues contribute the majority of the overall receptor-binding strength, and that the peptide-binding motif derived from the GlyR β subunit displays the highest gephyrin-binding potency. GlyR and GABA A R co-localization and agonist co-transmission were reported earlier [39] , [40] . It was shown that up to 35% of all GlyRs co-localize with GABA A Rs in the hypoglossal nucleus [39] and that 20–40% of all miniature postsynaptic currents recorded from respiratory glycinergic neurons are mixed miniature postsynaptic currents [40] that result from the co-release of GABA and glycine. The competition between GABA A Rs and GlyRs for an overlapping gephyrin-binding site, as shown here, suggests an interdependence of their clustering as well as their transport to the synapse. Major determinants of the competition would be the ratio of free receptor-binding sites in gephyrin and, among the gephyrin-binding receptor subunits, the gephyrin-binding subunit number within a pentameric receptor and the post-translational modifications of the respective motifs within these subunits [20] , [41] . Although GABA A R transport remains poorly characterized, GlyRs were shown to be retrogradely co-transported with gephyrin by the dynein motor complex via an interaction of the dynein light chain with the central linker of gephyrin [42] . If GABA A Rs would rely on the same pathway for their retrograde transport, both inhibitory receptor families would also compete for a common transport pathway, thus further intertwining their presence at inhibitory synapses. Finally, a recent study of the ultrastructure of spinal cord inhibitory synapses suggested that the GABA A R/GlyR competition for gephyrin-binding sites is regulated in an activity-dependent manner [23] . Overall, the GephE-peptide structures display a high similarity. However, two out of eight peptide chains in the GephE–peptide complexes derived from the orthorhombic and hexagonal space groups exhibit obvious differences in the orientation of GABA A R Tyr375 ( Supplementary Fig. 3 ). We find that these changes are due to crystal contacts with a neighbouring symmetry-related molecule and therefore do not indicate a difference between the two receptor-binding sites within a GephE dimer as suggested earlier [38] . Accordingly, our structures clearly support the view that both receptor-binding sites within a single GephE dimer are identical and hence are occupied in a non-cooperative manner. Our structural analysis demonstrates that the C-terminal halves of the GlyR and GABA A R gephyrin-binding core regions interact differently with gephyrin and occupy partially non-identical binding surfaces. The analysis of the chimeric peptide variants demonstrated that the C-terminal regions are crucial for the binding event by exhibiting an important enhancing effect. Furthermore, the structural and thermodynamic dissections revealed that the side chain interactions of GABA A R α3 residues Thr373, Thr374 and Tyr375 within this C-terminal receptor region are of major importance. Particularly, Tyr375, which is conserved among the α1, α2 and α3 GABA A R subunits, engages in critical hydrophobic interactions. Based on the sequence similarity of the gephyrin-binding region of the GABA A R α3 and α1 subunits and a previous mutagenesis study [18] , the gephyrin-binding interface of the GABA A R α1 subunit can be predicted ( Supplementary Fig. 7 ). The fact that different receptor subunits target gephyrin with unique binding motifs, which nonetheless engage in tight and specific interactions, allows for a subunit-specific post-translational regulation of this interaction. To this end, our study provides a possible structural explanation for the previously described regulation of GABAergic transmission by the extracellular signal-regulated kinases/mitogen-activated protein kinases pathway mediated by phosphorylation of GABA A R α1 Thr345, which is conserved within the gephyrin-binding site of GABA A R α1–3 and corresponds to GABA A R α3 Thr373 ( Supplementary Fig. 7 ) [43] . Furthermore, we provide a structural framework for future functional studies of phosphorylations at GABA A R α3 Thr374 and Tyr375 and their corresponding GABA A R α1 and α2 residues, which are phosphorylated in vivo [44] , [45] . It can be assumed that post-translational modifications of these residues modulate the gephyrin-GABA A R affinity, and hence, the residence time at the synapse in a similar manner as reported for the protein kinase C-mediated phosphorylation of GlyR β Ser399 (ref. 41 ). In contrast to glutamate receptors for which bacterial homologues have been identified, no GlyR-related receptors have been identified in bacteria. Furthermore, GlyRs are also absent from invertebrates [46] and, in agreement with this observation, only those residues that are required for the receptor interaction are conserved among gephyrin proteins from vertebrates [10] . In contrast, GABA A R α subunit-related proteins have been identified in invertebrates [46] and, in order to decipher how the gephyrin-binding motif evolved within the GABA A R family, we compared the corresponding sequences ( Supplementary Fig. 8 ). Similar to the gephyrin-binding motif of GlyRs, only vertebrate GABA A Rs, but not invertebrate GABA A Rs, contain a largely conserved gephyrin-binding sequence. This suggests that gephyrin-mediated GABA A R clustering evolved later than gephyrin-mediated GlyR clustering and that both motifs evolved independently. As major mediators of fast synaptic inhibition GABA A Rs are clinically relevant drug targets, and molecules that uncouple the central receptor-scaffold interaction at post-synaptic sites would therefore provide a powerful pharmacological tool with a possible therapeutic relevance. This principle has been demonstrated for the interaction between the N -methyl- D -aspartate-type glutamate receptors and the scaffolding postsynaptic density protein 95 (PSD-95), which has been targeted by peptide-based inhibitors [47] , [48] , [49] , [50] , [51] , [52] . This approach has shown great promise both as a pharmacological tool [51] , [53] and, in particular, in the development of therapeutically relevant compounds [54] , [55] . We therefore propose that conceptually similar molecules could be used to interfere with the receptor-scaffold interactions in vivo to modulate GABAergic and/or glycinergic transmission. Molecules that bind the universal N-terminal receptor-binding site with high affinity could be used as competitive inhibitors of gephyrin-mediated synaptic GlyR and GABA A R clustering. In addition, the described alternative receptor recruitment of GABA A Rs versus GlyRs by gephyrin, could form the basis for the development of subunit-specific modulators of either GABAergic or glycinergic transmission. Peptide synthesis, purification and characterization Apart from four chimeric peptides, which were purchased as lyophilized powder from Genscript, peptides were synthesized using Fmoc solid phase peptide synthesis. Preparative HPLC was performed on an Agilent 1100 system using a C18 reverse phase column (Zorbax 300 SB-C18, 21.2 × 250 mm 2 ) with a linear gradient of the binary solvent system of 0.1% trifluoroacetic acid in H 2 O/acetonitrile (ACN; A: 95:5 and B: 5:95) with a flow rate of 20 ml min −1 . Analytical HPLC was performed on an Agilent 1100 system with a C18 reverse phase column (Zorbax 300 SB-C18 column, 4.6 × 150 mm 2 ), a flow rate of 1 ml min −1 , and a linear gradient of the binary solvent system of 0.1% trifluoroacetic acid in H 2 O/ACN (A: 95:5 and B: 5:95). Mass spectra were obtained with an Agilent 6410 Triple Quadrupole Mass Spectrometer instrument using electron spray ionization coupled to an Agilent 1200 HPLC system (electrospray ionization–liquid chromatography/ mass spectrometry (ESI-LC/MS)) with a C18 reverse phase column (Zorbax Eclipse XBD-C18, 4.6 × 50 mm), autosampler and diode-array detector using a linear gradient of the binary solvent system of 0.1% formic acid in H 2 O/ACN (A: 95:5 and B: 5:95) with a flow rate of 1 ml min −1 . During ESI-LC/MS analysis, evaporative light scattering traces were obtained with a SedereSedex 85 Light Scattering Detector. The identity of all tested compounds was confirmed by ESI-LC/MS ( Supplementary Table 3 ), which also provided purity data (all >90%; ultraviolet and evaporative light scattering detection). All used peptides were water soluble at neutral pH in the millimolar range. Protein expression and purification GephE (gephyrin P1 splice variant residues 318–736) as well as residues 378–425 of the large cytoplasmic loop of the GlyR β subunit (β49) were expressed in E. coli BL21 (DE3) (Stratagene) as an intein fusion proteins with a chitin-binding domain for affinity purification [9] . Cells were grown in lysogeny broth medium at 30 °C and induced with 0.5–1 mM isopropyl-β-thiogalactoside at a cell density A 600 of 0.5–1. Cells were collected after 4 h (Intein-GlyR) or 20 h (GephE-Intein) by centrifugation (4,000 g ), resuspended in lysis buffer (50 mM Tris/HCl, pH 8.0, 500 mM NaCl) and passed through a cell disruptor (Constant Systems). Cell debris was removed by centrifugation (70,000 g ). Proteins were purified at room temperature (RT) using a chitin column according to the instructions of the IMPACT-TWIN protein expression and purification system (New England Biolabs). Cleavage of GephE from the N-terminal intein fusion was induced by a pH and temperature shift (100 mM NaCl, 20 mM Tris/HCl, 5 mM DTT, 1 mM EDTA, pH 6, 25 °C) and subsequent incubation for 48 h. Cleavage of β49 from the intein was accomplished by incubation with 100 mM DTT for 24 h. Protein containing fractions were collected, concentrated and applied to a 26/60 Superdex 200 size exclusion column (Amersham Biosciences) equilibrated with buffer (10 mM Tris/HCl, pH 8.0, 250 mM NaCl, 1 mM β-mercaptoethanol). Pure fractions were pooled, concentrated using Vivaspin 3 kDa molecular weight cutoff centrifugal filter devices (Sartorius Stedim Biotech) to 1–100 mg ml −1 , flash-frozen in 0.5 ml aliquots and stored at −80 °C. Protein conjugation for chemiluminescence detection Purified GephE was conjugated with HRP (Sigma-Aldrich) to enable its detection by chemiluminescence. The procedure is based on earlier reports [56] . In brief, 5 mg of lyophilized HRP were dissolved in 1 ml conjugation buffer (50 mM Na 2 CO 3 , pH 8.0). After incubation with 1 ml of 50 mM NaIO 4 for 30 min and 1 ml of 160 mM ethylene glycol for 1 h, the reaction mixture was dialysed against 10 mM Na 2 CO 3 , pH 9.5 at 4 °C overnight. 5 mg of GephE were added to the dialysed activated HRP containing solution and after incubation for 3 h, 5 mg of NaBH 4 were added and the reaction was stirred for another 3 h at 4 °C. After dialysis against SEC-buffer (10 mM Tris/HCl pH 8.0, 250 mM NaCl, 1 mM β-mercaptoethanol), the solution was centrifuged for 5 min at 10,000 g and the supernatant was applied to a 26/60 Superdex 200 size exclusion column (Amersham Biosciences) equilibrated with SEC-buffer. Pure fractions of the GephE-HRP-conjugate were identified via SDS–polyacrylamide gel electrophoresis and pooled according to chemiluminescence and concentrated using Vivaspin 3 kDa molecular weight cutoff centrifugal filter devices (Sartorius Stedim Biotech) to 1 mg ml −1 , flash-frozen in 0.1 ml aliquots and stored at −80 °C. Peptide array-based analysis The wild-type GABA A R α3 peptide ( 369 TFNIVGTTYPINLAK 384 ) and its respective Ala-variants were purchased from Intavis AG in a CelluSpot format. After rinsing of the peptide array slides with TBS (50 mM Tris, 150 mM NaCl, pH 7.6) and 0.05% Tween-20 (TBST) for 5 min, the peptide array was incubated with HRP-conjugated GephE (1 μM) in blocking buffer (TBST+5% nonfat dry milk) for 5 h at RT. After extensive washing, bound GephE-HRP-conjugate was detected by chemiluminescence using the Amersham ECL Prime Western Blotting Detection Reagent (GE Healthcare) using the chemiluminescent bio-imaging system MicroChemi (DNR Bio-imaging Systems). The resulting dot-blots were analysed using the array analyse software (Active Motif). Three peptide array duplicates were used to calculate the average spot densities and their rms deviations. Preparation of whole brain lysates After cervical dislocation, whole brains from 54-week-old C57Bl/6J male mice were removed from the scull and rapidly homogenized in 1 ml lysate buffer (20 mM HEPES, 100 mM K-acetate, 40 mM KCl, 5 mM EGTA, 5 mM MgCl 2 , 5 mM DTT, 1 mM PMSF, 1% Triton X, protease inhibitor Roche complete, pH 7.2) per 200 mg using a pistol homogenizer (8 strokes at 900 r.p.m.). The homogenate was centrifuged at 10,000 g for 15 min. Subsequently, the supernatant was removed and aliquots were flash-frozen in liquid nitrogen and stored at −80 °C. Covalent immobilization of peptides GABA A R α3 peptide fragments with an additional C-terminal Cys ( 368 FNIVGTTY 375 C, 368 FNIVGTTYP 376 C, 368 FNIVGTTYPI 377 C, 368 FNIVGTTYPIN 378 C) were coupled to UltraLinkIodoacetyl Gel (Thermo Scientific) according to the protocol of the manufacturer: the peptides were dissolved in coupling buffer (50 mM Tris, 5 mM EDTA, pH 8.5) at a concentration of 1 mM and incubated for 2 h at RT with UltraLink beads, which had been washed and equilibrated with coupling buffer before. After removing excess peptides, the UltraLink beads were subjected to 1 mM cysteine for 2 h to quench possible unreacted iodoacetyl groups. The resin was washed three times and equilibrated with 1 M NaCl and stored at 4 °C. Pull-down and western blot detection The resin with the immobilized peptides was incubated with brain lysate for 1 h at 4 °C. After three washing steps with lysate buffer, the beads were boiled with Laemmli buffer containing 10% SDS. Subsequently, the supernatant was applied to an SDS–polyacrylamide gel electrophoresis followed by western blotting against gephyrin using the mAb7a antibody [37] (Synaptic Systems) at a dilution of 1:500. Peptide and protein concentration determination The concentration of the GephE stock-solution was determined by amino-acid analysis and aliquots of an identical stock were used for all experiments to ensure comparability of all experiments and rule out effects of protein activity, degradation, concentration determination and aggregation. Peptide stocks were prepared by weighing the lyophilized powders. All ITC titrations displayed stoichiometries between 0.96 and 1.04, thus, demonstrating a high accuracy of the measured concentrations and comparability of the results. Isothermal titration calorimetry The experiments were performed using an ITC200 (MicroCal) at 25 °C and 1,000 r.p.m. stirring and designed so that c -values were generally within 0.5–100 ( c -value= K A × [protein] × N with K A , equilibrium association constant; [protein], protein concentration; N , stoichiometry). Specifically, 40 μl of a solution containing 1–3 mM of the peptide were titrated into the 200 μl sample cell containing 25–100 μM GephE. In each experiment, a volume of 1–2 μl of ligand was added at a time resulting in 20–40 injections and a final molar ratio between 1:3 and 1:6. Ligand-to-buffer titrations were carried out in an analogous manner, so that the heat produced by injection, mixing and dilution could be subtracted. The binding enthalpy was directly measured, whereas the dissociation constant ( K D ) and stoichiometry ( N ) were obtained by data analysis using the Origin software (OriginLab). Measurements were conducted at least three times and are given as mean values with the resulting standard deviations. Protein complex crystallization and X-ray data collection Complexes of GephE and peptides α11 WT and α11 SL were prepared by mixing both in a 1:5 (protein/peptide) molar ratio followed by incubation at 4 °C for 15 min. The complexes were crystallized by the hanging drop vapour diffusion method at 20 °C at a concentration of 10 mg ml −1 in the presence of 0.2 M calcium acetate, 0.1 M MES, pH 6, and 6–10% isopropanol as precipitant. Both complexes were also crystallized at 4 °C at a concentration of 2.5 mg ml −1 with 0.1 M Tris, pH 7.5, and 21–27% PEG4000 as precipitant. The crystals were transferred to the respective mother liquor solution containing 25% glycerol as cryoprotectant and flash frozen in liquid nitrogen. The data sets were collected at beam lines ID14–4 and ID 23-2 at the ESRF, Grenoble ( Table 1 ). Structure determination and refinement The data sets were indexed and integrated with iMosflm [57] or XDS [58] , further scaling and merging were done by using the CCP4 suite [59] . The structures were solved by molecular replacement with Phaser [60] using 2FU3 as initial model [10] . Refinements were carried out with PHENIX [61] and Refmac5 (ref. 59 ). The crystals grown at 4 °C belonged to space group P2 1 2 1 2 and diffracted to a resolution of 2.7 Å, the crystals grown at 20 °C to space group P6 1 , which diffracted only to low resolutions of 3.6–4.1 Å. For low-resolution refinement, the 1.7-Å resolution apo-E domain structure (PDB: 4PDO) was used as reference model. Figures involving molecular representations were prepared using PyMol ( http://www.pymol.org ). How to cite this article: Maric, H. M. et al. Molecular basis of the alternative recruitment of GABA A versus glycine receptors through gephyrin. Nat. Commun. 5:5767 doi: 10.1038/ncomms6767 (2014). Accession codes: The coordinates have been deposited in the Protein Data Bank with the following codes: 4TK1 (orthorhombic) and 4TK2 (hexagonal) for GephE-α11 WT , 4TK3 (orthorhombic) and 4TK4 (hexagonal) for GephE-α11 SL structures.